New loci for body fat percentage reveal link between adiposity and cardiometabolic disease risk To increase our understanding of the genetic basis of adiposity and its links to cardiometabolic disease risk, we conducted a genome-wide association meta-analysis of body fat percentage (BF%) in up to 100,716 individuals. Twelve loci reached genome-wide significance ( P <5 × 10 −8 ), of which eight were previously associated with increased overall adiposity (BMI, BF%) and four (in or near COBLL1/GRB14 , IGF2BP1 , PLA2G6 , CRTC1 ) were novel associations with BF%. Seven loci showed a larger effect on BF% than on BMI, suggestive of a primary association with adiposity, while five loci showed larger effects on BMI than on BF%, suggesting association with both fat and lean mass. In particular, the loci more strongly associated with BF% showed distinct cross-phenotype association signatures with a range of cardiometabolic traits revealing new insights in the link between adiposity and disease risk. Large-scale meta-analyses of genome-wide association studies (GWAS) for adiposity traits and obesity risk have identified at least 160 loci that contribute to body weight and fat distribution in adults and children of diverse ancestry [1] , [2] , [3] , [4] , [5] , [6] , [7] , [8] , [9] , [10] , [11] , [12] , [13] , [14] , [15] , [16] , [17] , [18] , [19] , [20] . Studies of overall adiposity, assessed by body mass index (BMI), have mainly implicated genes that provide support for a role of the central nervous system (CNS) in obesity susceptibility [1] , [2] , [3] , [4] , [5] , [6] , [10] , [19] , whereas genetic loci associated with body fat distribution, assessed by waist-to-hip ratio (WHR), seem enriched for genes involved in adipocyte metabolism [9] , [11] , [20] . Although these commonly studied adiposity traits are easily collected in large populations and thus allow statistically well-powered meta-analyses, they represent heterogeneous phenotypes, for example, people with the same BMI or WHR may vary in BF%, translating in differences in cardiometabolic risk [21] , [22] . To assess the genetic contribution to adiposity, we previously performed the first GWAS for BF% in nearly 40,000 individuals and identified two new loci (near IRS1 and SPRY2 ), not identified in earlier large-scale GWAS for BMI [13] . Follow-up analyses of these loci provided strong evidence for IRS1 to be involved in tissue-specific body fat storage and subsequent effects on cardiometabolic disease, such as type 2 diabetes (T2D) and coronary artery disease (CAD) [13] . While little is known about SPRY2 , the Spry1 homolog in mice has been implicated in adipose tissue differentiation [23] . Taken together, these loci for BF% pointed towards new mechanisms involved in adipocyte metabolism that differ from the BMI-associated loci that suggested a role for the CNS [13] , [19] . Here, we have extended our study to include more than 100,000 individuals and continue to discover novel genetic loci associated with BF% that have not been identified before for any of the commonly studied adiposity traits [1] , [2] , [3] , [4] , [5] , [6] , [7] , [8] , [9] , [10] , [11] , [12] , [13] , [14] , [15] , [16] , [17] , [18] , [19] , [20] . Through an in-depth integrative characterization, including cross-trait association analyses, expression quantitative trait loci (eQTL), pathway and network analyses, regulome analyses and transgenic drosophila models, we show that these loci provide new insights into the biology that underlies adiposity and related cardiometabolic health, by specifically highlighting peripheral physiological mechanisms. 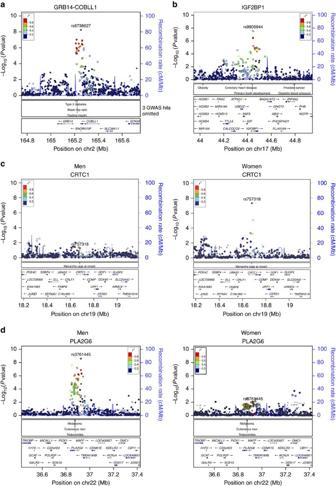Figure 1: Regional plots of the four newly identified loci that reached genome-wide significant association with body fat percentage. Regional plots of the four newly identified loci that reached genome-wide significant association with body fat percentage in all-ancestry analyses, in men and women combined for theCOBLL1/GRB14andIGF2BP1loci (a,b), and separately for theCRTC1andPLA2G6(c,d). Each symbol represents the significance (Pvalue on a −log10 scale) of a SNP with BF% as a function of the SNP’s genomic position (NCBI Build 36). For each locus, the index SNP is represented in the purple colour. The colour of all other SNPs indicates LD with the index SNP (estimated by CEUr2from the HapMap Project data Phase II CEU). Recombination rates are also estimated from International HapMap Project data, and gene annotations are obtained from the UCSC Genome Browser. GWAS catalogues SNPs withPvalue <5 × 10−8are shown in the middle panel. Different shapes denote the different categories of the SNPs: up-triangle for framestop or splice SNPs, down-triangle for nonsynonymous SNPs, square for coding or untranslated region (UTR) SNPs; star for SNPs in tfbscons region, square filled with ‘X’ symbol for SNPs located in mcs44placental region and circle for SNPs with no annotation information. Analyses in >100,000 individuals identify 12 loci for BF% In our primary meta-analysis, we combined results of genetic associations with BF% for up to 100,716 individuals from 43 GWAS ( n up to 76,137) and 13 MetaboChip studies ( n up to 24,582), predominantly of European ancestry ( n up to 89,297), but also of non-European ancestry ( n up to 11,419) populations ( Supplementary Table 1 and Supplementary Fig. 1 ). As women have on average a higher BF% than men, we also stratified meta-analyses by sex ( n men up to 52,416; n women up to 48,956). In secondary meta-analyses, we combined data from European-ancestry populations only ( n up to 89,297; n men up to 44,429; n women up to 45,525) to reduce genotypic and phenotypic heterogeneity that may have been introduced in the overall analyses by combining diverse ancestries. In our primary meta-analysis of men and women combined, single-nucleotide polymorphisms (SNPs) in 10 independent loci reached genome-wide significance (GWS, P <5 × 10 −8 ; Table 1 and Supplementary Fig. 2 ), including the three loci that we identified before [13] . Two additional loci, near PLA2G6 and in CRTC1 , were identified in men-specific and women-specific analyses, respectively ( Table 1 and Supplementary Fig. 3 ). The European-ancestry-only analyses revealed the same loci, but no additional ones ( Supplementary Tables 4–6 , Supplementary Figs 4 and 5 ). We did not identify evidence of secondary signals at any of the 12 loci. Table 1 Loci reaching genome-wide significance ( P <5 × 10 −8 ) for body fat percentage in all ancestry analyses, sorted according to significance in the overall analysis. Full size table Two (near IRS1 and SPRY2 ) of the 12 loci had been first identified in our previous genome-wide screen for BF% (ref. 13 ), and six loci (in/near FTO , MC4R , TMEM18 , TOMM40/APOE , TUFM / SH2B1 and SEC16B ) had been first reported for association with BMI [1] , [2] , [3] , [4] , [5] , [6] , [10] . Four of the 12 loci, in or near COBLL1/GRB14 , IGF2BP1 , PLA2G6 and CRTC1 , have not been associated with an overall adiposity trait (such as BMI, BF%, obesity risk) before ( Fig. 1 and Supplementary Fig. 6 ). 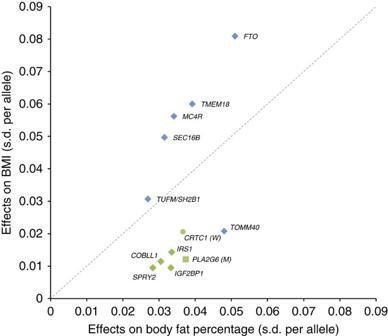Figure 2: Comparison of effects of the 12 loci on body fat percentage (xaxis) and on BMI (yaxis). Both outcomes (BMI and BF%) were inverse normally transformed (mean 0, s.d. 1) such that effects sizes are at the same scales and directly comparable. Effect sizes for BMI were obtained from Lockeet al.19. The allele effects for thePLA2G6(square) andCRTC1(round) loci were derived, respectively, from the men- and women-based meta-analyses. Six loci had first been identified for BMI (blue), whereas six others were first identified for BF% (green). Of note, the COBLL1/GRB14 locus was previously established as a locus for body fat distribution independent of overall adiposity, assessed by WHR adjBMI [11] , and the CRTC1 locus has been first reported for its association with age at menarche [24] ( Table 2 , Supplementary Table 7 , See also ‘Cross-phenotype association’ section). Figure 1: Regional plots of the four newly identified loci that reached genome-wide significant association with body fat percentage. Regional plots of the four newly identified loci that reached genome-wide significant association with body fat percentage in all-ancestry analyses, in men and women combined for the COBLL1/GRB14 and IGF2BP1 loci ( a , b ), and separately for the CRTC1 and PLA2G6 ( c , d ). Each symbol represents the significance ( P value on a −log10 scale) of a SNP with BF% as a function of the SNP’s genomic position (NCBI Build 36). For each locus, the index SNP is represented in the purple colour. The colour of all other SNPs indicates LD with the index SNP (estimated by CEU r 2 from the HapMap Project data Phase II CEU). Recombination rates are also estimated from International HapMap Project data, and gene annotations are obtained from the UCSC Genome Browser. GWAS catalogues SNPs with P value <5 × 10 −8 are shown in the middle panel. Different shapes denote the different categories of the SNPs: up-triangle for framestop or splice SNPs, down-triangle for nonsynonymous SNPs, square for coding or untranslated region (UTR) SNPs; star for SNPs in tfbscons region, square filled with ‘X’ symbol for SNPs located in mcs44placental region and circle for SNPs with no annotation information. Full size image Table 2 Cross-phenotype associations: associations signatures of 12 established body fat percentage loci for anthropometric and cardiometabolic traits through look-ups in large-scale genetics consortia. Full size table Effect sizes and explained variance Index SNPs in the 12 established loci increase BF% by 0.024 to 0.051 s.d. per allele (equivalent to 0.16 to 0.33% in BF%, Table 1 , Fig. 2 ). Given the high correlation between BF% and BMI, the BF% increasing alleles of each of the 12 loci are associated with increased BMI ( Fig. 2 , Table 2 , and Supplementary Table 7 ). However, loci that had been previously identified for BMI, have larger effects (expressed in s.d. per allele) on BMI than on BF%, except the TOMM40/APOE locus, which has a substantially more pronounced effect on BF% than on BMI [25] ( Fig. 2 ). The TOMM40/APOE locus, together with the loci previously ( IRS1 and SPRY2 ) and newly ( COBLL1 / GRB14 , IGF2BP1 , PLA2G6 and CRCT1 ) identified for BF% all have larger effects on BF% than on BMI ( Fig. 2 ). This division based on effect sizes, illustrated in Fig. 2 , suggests that IRS1, SPRY2, COBLL1/GRB14, TOMM40/APOE, IGF2BP1, PLA2G6 and CRTC1 affect adiposity in particular, which is not fully captured by BMI (which represents both lean and fat mass). Figure 2: Comparison of effects of the 12 loci on body fat percentage ( x axis) and on BMI ( y axis). Both outcomes (BMI and BF%) were inverse normally transformed (mean 0, s.d. 1) such that effects sizes are at the same scales and directly comparable. Effect sizes for BMI were obtained from Locke et al. [19] . The allele effects for the PLA2G6 (square) and CRTC1 (round) loci were derived, respectively, from the men- and women-based meta-analyses. Six loci had first been identified for BMI (blue), whereas six others were first identified for BF% (green). Full size image Of the 12 loci, four showed significant sex-specific effects. For the loci near IRS1 and PLA2G6, the effect in men was twice as large as in women, whereas for the TMEM18 and CRTC1 loci the effect was two- to threefold larger in women than in men ( Table 1 ). As the European-ancestry-only populations represent the vast majority (90%) of the total sample, effects sizes from European only and all-ancestry analyses were similar ( Supplementary Tables 5 and 8 ). In aggregate, the 12 loci explained 0.58% of the variance in BF% in men and women combined. Because of the sex-specific effects of four loci, the explained variance was slightly higher, when estimated in men (0.62%) and women (0.61%) separately. Individually, the FTO locus explained the most variance of all identified loci (0.12%) ( Table 1 ). Cross-phenotype association with cardiometabolic traits To gain insight in how the BF% loci affect anthropometric and cardiometabolic traits and comorbidities, we performed look-ups in the most recent large-scale GWAS meta-analyses from the GIANT (Genetic Investigation of ANthropometric Traits) consortium (WHR adjBMI and height) [20] , [26] , the SAT-VAT consortium (abdominal visceral adipose tissue (VAT) and subcutaneous adipose tissue (SAT)) [27] , the LEPgen consortium (circulating leptin), the GLGC (high-density lipoprotein cholesterol (HDL-C), low-density lipoprotein cholesterol (LDL-C) and triglycerides (TG)) [28] , the MAGIC (fasting glucose and fasting insulin) [29] , DIAGRAM (T2D) [30] and CARDIoGRAMplusC4D (CAD) [31] . To account for multiple testing, associations were considered statistically significant if P values were <5.2 × 10 −4 (Bonferroni-corrected P =0.05/96 (12 SNP * eight trait groups)). Associations with anthropometric and adiposity traits . The BF% increasing alleles for 11 of the 12 loci were associated with increased circulating leptin levels ( P binomial =0.006), of which four reached statistical significance and another four were nominally significant ( Table 2 , Supplementary Table 7 ). These results are consistent with the notion that leptin is secreted by adipocytes proportional to adipose tissue mass. The BF% increasing alleles of all 12 loci were associated with increased SAT and VAT ( P binomial =0.0005), two ( FTO and TMEM18 ) of which reached significance for association with SAT, and two ( FTO and TOMM40/APOE ) with VAT. The BF% increasing allele of the locus near IRS1 was associated with a lower VAT/SAT ratio, indicative of a proportionally greater subcutaneous than visceral fat storage, as we have shown previously [13] ( Table 2 , Supplementary Table 7 ). As expected, most of the identified BF% loci showed no association with WHR adjBMI , as this trait, because of the adjustment for BMI, does not correlate with overall adiposity. Nevertheless, associations with WHR adjBMI for two loci ( COBLL1/GRB14 and TOMM40/APOE ) did reach statistical significance. The COBLL1/GRB14 locus was previously identified as a WHR adjBMI locus [11] . We show that it is the BF% increasing allele that is associated with lower WHR adjBMI , suggestive of a preferential gluteal rather than abdominal fat storage. Although the COBLL1/GRB14 association with WHR adjBMI is five times stronger in women than in men [11] , we observed no sex difference for association with BF% ( Table 1 ). For the TOMM40/APOE locus, it is the BF% increasing allele that is also associated with increased WHR adjBMI , suggesting that the TOMM40/APOE locus increases abdominal and overall fat accumulation, at least in part, in an additive and independent manner. Furthermore, the BF% increasing allele was also significantly associated with increased VAT ( Table 2 , Supplementary Table 7 ) and liver fat storage ( P =3.4 × 10 −4 , n =5,550, Methods section). SNPs in three loci ( MC4R , PLA2G6 and IGF2BP1 ) showed significant association with height, two of which ( PLA2G6 and IGF2BP1 ) have not been reported in large GWAS studies before. Similar to the MC4R locus, the BF% increasing allele of the PLA2G6 (rs3761445) was associated with greater adult height ( P =6.7 × 10 −5 ; Table 2 , Supplementary Table 7 ). Following up this variant in data from the Early Growth Genetics Consortium, we found that the BF% increasing allele was associated with higher birth weight ( P =0.003, n up to 26,836; ref. 32 ) and greater prepubertal height ( P =0.007, n =13,948; ref. 33 ), yet not with growth during or timing of puberty ( Supplementary Table 10 ) [33] . In contrast, the BF% increasing allele in IGF2BP1 (rs9906944) was associated with shorter height ( Table 2 , Supplementary Table 7 ), a cross-phenotype association pattern that is consistent with the effects of the GH/IGF1 axis [34] . SNPs in IGF2BP1 , in linkage disequilibrium (LD) with rs9906944 ( r 2 EUR =0.47), have been previously implicated with primary tooth development in infancy [35] . Consistently, the BF% increasing allele of IGF2BP1 (rs9906944) showed association with a later eruption of the first tooth ( β =0.16 months per allele; P =3.1 × 10 −8 ) and reduced number of teeth at 1 year ( β =−0.14 number of teeth at age 1 year per allele; P =1.1 × 10 −7 ; ref. 35 ). Even though this suggests a role in maturation, we found no evidence for association with pre-pubertal height or pubertal growth and timing ( Supplementary Table 10 ) [33] or age at menarche ( β =0.01 age of menarche (years) per allele; P =0.11; ref. 24 ). Although this locus harbours a number of genes, data in rodents suggest that IGF2BP1 might be a potential candidate gene driving the associations observed here, as Igf2bp1 knockout mice demonstrate fetal and postnatal growth retardation [36] . Taken together, alleles of each of the 12 loci are associated with increased BF%, yet their associations with other anthropometric traits differ, which in turn might result in varying impacts on cardiometabolic health. Associations with cardiometabolic traits . Although phenotypic correlations observed in epidemiological studies have shown that increased adiposity is associated with increased cardiometabolic risk, the BF% increasing alleles of identified loci do not always associate with poorer health outcomes ( Table 2 and Supplementary Table 11 ). For some loci, the BF% increasing allele may even have significant protective effects, as we have shown previously for the locus near- IRS1 (ref. 13 ). For the loci in/near FTO, MC4R, TMEM18, TUFM/SH2B1 and SEC16B, which were all five previously established for BMI, the observed cross-phenotype associations with cardiometabolic traits are generally directionally consistent with the phenotypic correlations. Specifically, their BF% increasing allele is typically associated with an unfavourable lipid profile and increased insulin resistance ( Table 2 , Supplementary Tables 12 and 13 ). These cross-phenotype associations translate in increased risk of T2D and CAD and higher CRP levels, at least for the FTO, TMEM18 and MC4R loci ( Fig. 2 , Table 2 , Supplementary Tables 9,12 and 13 ). For the remaining seven loci, which all have a larger effect on BF% than on BMI ( Fig. 2 ), the cross-phenotype associations are not always consistent with the phenotypic correlation between BF% and cardiometabolic traits. For example, the COBLL1/GRB14 locus was previously identified for its association with fasting insulin [29] , TG [37] , HDL-C [37] and,T2D risk [30] ( Table 2 , Supplementary Tables 12 and 13 ). However, we show for the first time that it is the BF% increasing allele that is associated with a protective effect on cardiometabolic health; that is, with significantly lower TG levels and higher HDL-C levels, and a reduced risk of T2D ( Table 2 , Supplementary Tables 12 and 13 ). This association signature of the COBLL1 / GRB14 locus is consistent with the observation that its BF% increasing allele is associated with a lower WHR adjBMI , corresponding to a proportionally lower abdominal and higher gluteal fat accumulation and, at nominal significance, with SAT but not with the metabolically more harmful VAT. The COBLL1 / GRB14 association signature is similar to that of the near- IRS1 locus ( Table 2 , Supplementary Tables 12 and 13 ), and suggest that the beneficial cardiometabolic effects of the loci near COBLL1/GRB14 and IRS1 might be mediated through a favourable influence on body fat distribution, despite increased adiposity. The BF% increasing allele of rs6857 near TOMM40 / APOE is significantly associated with increased overall adiposity (BMI), abdominal adiposity (WHR adjBMI ), visceral adipose tissue (VAT) and liver fat storage, which may be mediating the nominally significant association with increased fasting glucose and risk of T2D ( Table 2 and Supplementary Table 13 ). However, most notably, the BF% increasing allele was also highly significantly associated with a favourable lipid profile and reduced risk of CAD ( Table 2 and Supplementary Table 12 ). The associations with lipid levels seem to be only partially driven by the nearby APOE locus for which previously highly significant associations with LDL-C [37] , CRP [38] (both rs4420638), HDL-C and TG (rs439401; ref. 37 ) levels have been reported ( Supplementary Fig. 7 ). These two SNPs (rs4420638, rs439401) are in low LD with each other ( r 2 EUR =0.13, D′ EUR =0.96), and with the here-identified TOMM40 -rs6857 ( r 2 EUR =0.39, D′ EUR =0.72 and r 2 EUR =0.06, D′ EUR =0.77, respectively). Although the APOE -rs4420638 allele shows evidence of association with BF% ( P =3.9 × 10 −5 ), the association is completely abolished ( P =1.00) after conditioning for TOMM40 -rs6857 ( Supplementary Table 14 ). The APOE -rs439401 SNP, previously associated with HDL-C levels, was not associated with BF% ( P =0.72). Conversely, the TOMM40 -rs6857 associations with TG ( P =4.5 × 10 −19 ; P conditional =3.6 × 10 −5 ) and HDL-C ( P =2.6 × 10 −17 ; P conditional =8.4 × 10 −14 ) remain significant after conditioning for the lipid-associated APOE SNPs (rs4420638, rs439401), whereas its association with LDL-C ( P =5.1 × 10 −110 ; P conditional =0.97) is completely abolished after adjusting for the APOE- rs4420638 ( Supplementary Table 14 ). Taken together, these observations show that associations of TOMM40 -rs6857 are independent from the HDL-C and TG-associated APOE -rs439401 and partially independent from the LDL-C-associated APOE- rs4420638 ( Supplementary Table 14 ). Another SNP (rs2075650) in this region, in high LD ( r 2 EUR= 0.77, D′ EUR =0.96) with the TOMM40 -rs6857 and associated with BF% ( P =1.4 × 10 −7 ), has been previously identified for its association with Alzheimer’s disease [39] , cognitive function [40] and ageing [41] , with the BF% increasing allele being associated with reduced risk of Alzheimer’s disease, slower cognitive decline and increased longevity. Although we do not observe association of IGF2BP1 -rs9906944 with circulating lipid levels or glycemic traits, interestingly, the BF% increasing allele is significantly associated with increased risk of T2D and CAD, and with higher CRP levels ( Table 2 , Supplementary Tables 9,12 and 13 ). The sex-specific effect of PICK1 / PLA2G6 -rs3761445 does not translate in sexual dimorphic associations with other traits ( Table 2 , Supplementary Tables 12 and 13 ). Interestingly, the BF% increasing allele is associated with a favourable lipid profile; in particular with lower TG levels ( P =8.1 × 10 −12 ) and higher HDL-C levels ( P =3.9 × 10 −6 , Supplementary Table 12 ), but no association with CAD risk was observed ( Supplementary Table 12 ). The PICK1 / PLA6G2 -rs3761445 is in moderate LD with SNPs identified before for nevus count (rs2284063, r 2 EUR =0.67, D′ EUR =0.90; ref. 42 ) and melanoma risk (rs738322, r 2 EUR =0.77, D′ EUR =0.98; refs 42 , 43 ). Consistently, the rs3761445 BF% increasing allele is associated with a lower number of cutaneous nevi (−0.067 nevi/allele, P =9.4 × 10 −6 ; ref. 43 ) and reduced melanoma risk (OR=0.86 per allele, P =5.3 × 10 −10 ; ref. 44 ). The BF% increasing allele of CRTC1 -rs757318, which showed a significantly stronger association in women than men, was not associated with any of the cardiometabolic traits in either sex-stratified or sex-combined results. Rs757318 is in moderate LD ( r 2 EUR =0.57, D′ EUR =1) with another CRTC1 SNP (rs10423674) that was previously established for age at menarche [24] and, consistently, also the rs757318 BF% increasing allele was significantly associated with earlier age at menarche ( β =−0.03 years per allele; P =2.4 × 10 −10 ; ref. 24 ). Functional annotation of genome-wide significant loci The causal genes and/or variants underlying most of the BF% associated loci remain unknown. For the 12 genome-wide significant loci, and also for putative loci ( P <1 × 10 −5 ), we used multiple complementary approaches to prioritize candidate genes and/or variants and to elucidate the mechanisms involved in body fat regulation. These approaches include identification of nearby coding variants or copy-number variants (CNVs), cis -eQTL analysis, epigenetic marker and functional regulatory genomic element analysis, pathway and tissue enrichment analysis, and a transgenic Drosophila model. Coding variants and CNV analysis . Among the 12 index SNPs, only rs4788099 near SH2B1 was in high LD with seven coding variants ( r 2 EUR >0.7) in nearby genes ( APOBR, SH2B1 and ATP2A1 ; Supplementary Table 15 , Methods section). Two of these seven variants were non-synonymous, of which, one, Thr484Ala (rs7498665) in SH2B1 , was in perfect LD with our index SNP. Thr484Ala shows a high degree of conservation, but was predicted to be functionally benign by PolyPhen and tolerated by SIFT. None of the other 11 index SNPs were in high LD with coding or CNVs. eQTL analysis . We examined cis -associations between each index SNP and gene expression of transcripts within 1 Mb-region flanking the respective SNP ( Supplementary Tables 16 and 17 , Methods section). As shown previously [13] , the BF% increasing allele of rs2943652 near IRS1 is associated with increased IRS1 expression in omental and subcutaneous fat. SNPs within the same locus (LD r 2 EUR >0.95) have also been shown to be associated with increased IRS1 expression in skeletal muscle [45] . We also identified significant ( P <1 × 10 −5 or 5% FDR) eQTLs for other BF% associated loci, even after conditioning for the most significant SNP-transcript association in the regions. The BF% increasing allele of COBLL1 / GRB14 -rs6738627 is associated with lower expression of GRB14, whereas there is no evidence of association with COBLL1 expression. The BF% increasing allele for PLA2G6 / MAFF -rs3761445 is associated with lower expression of MAFF and TMEM184B in omental and subcutaneous fat. TUFM / SH2B1- rs4788099 is associated with the expression of a number of genes, such as TUFM (blood), APOBR (blood), SBK1 (blood), SULT1A2 (omental and subcutaneous fat) and SH2B1 (omental fat). Epigenetic marker and functional regulatory genomic element analysis . We examined the overlap of 746 variants in LD ( r 2 CEU >0.70) with the 12 index SNPs with regulatory elements in brain, blood, liver, adipose and pancreatic islets from the ENCODE Consortium and Roadmap Epigenomic Projects ( Supplementary Table 18 ). Across loci, 179 (24%) variants showed evidence of being located in a regulatory element as defined by overlapping variants in two or more data sets from the same tissue ( Supplementary Table 19 ). Promoter variants, located within 2 kb of a transcription start site, overlapped with an average of 22 regulatory elements, while more distal variants (>2 kb) overlapped with an average of nine elements. Two of the distal variants with the greatest amount of regulatory overlap were rs4808844 and rs4808845 (43 and 41 elements, respectively; Supplementary Table 19 ). These variants are located 58 bp apart in intron 1 of CRTC1 and overlap evidence of open chromatin, histone marks that are characteristic of active transcription regulation and Pol2 binding ( Fig. 3a ). We found that rs4808844 was significantly associated ( P =0.036) with Pol2 binding signal strength ( Fig. 3b ). In addition, DNaseI hypersensitivity signal in this region has been shown to negatively correlate with CRTC1 and CRLF1 transcription levels across many cell types [46] . These data suggest that rs4808844 and rs4808845, both in high LD ( r 2 CEU =0.76 and 0.79, respectively) with our index SNP (rs757318), may influence the transcription of these and/or other nearby genes. 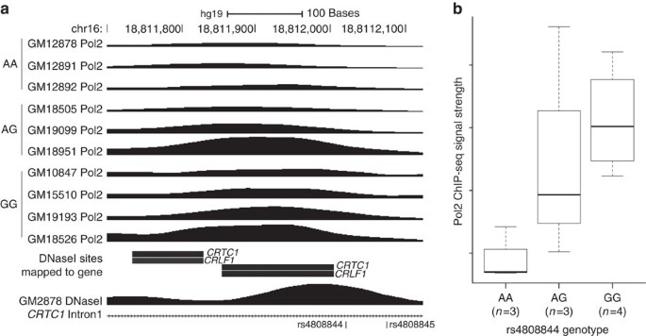Figure 3: Genotype influences Pol2 binding at rs4808844. (a) UCSC Genome browser track (hg19) of chromosome 16 displaying Pol2 binding signal in 10 lymphoblastoid cell lines (LCLs), grouped by genotype and correlations between DNaseI hypersensitivity and nearby gene transcription. (b) Binding signals from Pol2 ChIP-seq from 10 LCLs, grouped by genotype. Figure 3: Genotype influences Pol2 binding at rs4808844. ( a ) UCSC Genome browser track (hg19) of chromosome 16 displaying Pol2 binding signal in 10 lymphoblastoid cell lines (LCLs), grouped by genotype and correlations between DNaseI hypersensitivity and nearby gene transcription. ( b ) Binding signals from Pol2 ChIP-seq from 10 LCLs, grouped by genotype. Full size image We further characterized variants overlapping with regulatory elements at each of the 12 loci using RegulomeDB, and two loci stood out. In the TUFM-SH2B1 region, three SNPs (rs4788084, rs1074631 and rs149299) in LD ( r 2 CEU =0.82, 0.76 and 0.75, respectively) with rs4788099 are located in an EBF1-binding protein ChIP-seq signal in lymphoblastoid cells. In addition, rs4788084 is located within an EBF1-binding motif. EBF1 is involved in the thalamic axon projection into the neocortex [47] and the genetic variants around rs4788099 might affect the regulation of EBF1 of the nearby SH2B1 (ref. 48 ). In the PLA2G6/PICK1 region, rs4384 in LD with rs3761445 ( r 2 EUR =0.73) overlapped with more elements (50 elements in four tissues, Supplementary Table 19 ) than any other distal variant. This variant is located in a HEN1-binding motif with evidence of a DNase footprint in multiple cell types ( Supplementary Fig. 8 ). HEN1 is a transcription factor potentially involved in the CNS development [49] . Pathway, network and tissue-enrichment analysis . To test for enrichment and define pathways and networks between the genes harboured by the 12 GW-significant loci and 31 loci with putative evidence ( P <1 × 10 −5 ) of association with BF%, we applied a number of approaches (see Methods section). Neither DEPICT (data-driven enrichment prioritized integration for complex traits) [50] nor Ingenuity IPA identified pathways, tissues or networks that were significantly enriched among the genes across the 43 loci ( Supplementary Tables 20–22 ). Also, GRAIL (Gene Relationships Among Implicated Loci), which searches the published literature to identify relationships between genes, and DAPPLE (Disease Association Protein–protein Link Evaluator), which tests for protein–protein interactions, did not identify significant connection between any of the genes in the identified loci. Their limited power may be due to the relatively small number of loci identified in this meta-analyses or to limited knowledge related to adipogenesis [51] . Experimental follow-up of candidate genes in Drosophila We used Drosophila as a fast and inexpensive model to help prioritize which genes within the identified loci are the most likely candidates to underlie the observed associations. To gain first insights in the potential candidacy of the genes located within the 12 BF% associated loci, we performed a look-up in data from a genome-wide transgenic RNAi screen for fat content in adult Drosophila [52] . In that screen, whole-body TG, also in Drosophila the major lipid storage form, were used as a direct measure of fly adiposity upon activation of a heat shock-inducible Hsp70-GAL4 system. As such, transgenic fly lines were made to test the adiposity regulating potential of 10,489 of the ∼ 14,000 annotated Drosophila protein coding genes. Of the 80 genes located within a 1 Mb-window of each of the 12 index SNPs, 44 Drosophila orthologues were available, yet, 12 of these 44 transgenic RNAi fly lines were too weak to be screened. Of the remaining 32 fly lines, 15 fly lines had substantially lower (>2 s.d. less) whole-body TG than the wild-type flies, whereas five fly lines showed higher TG (>2 s.d. more) ( Supplementary Table 23 ). Next, we selected one to three candidate genes within each of the 12 loci based on their potential role in adipocyte metabolism. We knocked down their corresponding orthologues in Drosophila that were subsequently exposed to a high-sugar diet ( Supplementary Table 24 ), as described before [53] . Both Drosophila experiments pinpoint the SPRY2 (or sty ) as the potential causal gene within the locus; that is, knockdown flies for sty have significantly lower whole-body TG levels than wild-type flies. While the genome-wide transgenic RNAi screen pointed towards the CRTC1 gene in the CRTC1 locus, we could not confirm a role for CRTC1 in the knockdown experiment. Established loci and body fat percentage The most recent GWAS meta-analysis for BMI, including nearly 340,000 individuals, identified 97 loci that reached GWS [19] . Each of the 97 BMI-associated SNPs showed directionally consistent association with BF% ( P binomal <1 × 10 −4 ), 71 of which also reached nominal statistical significance ( Supplementary Table 25 ). One of the reasons for the non-significance for the remaining loci might be insufficient power as the current final meta-analysis sample size for BF% was only one-third of that for BMI. Of the 12 loci previously identified through GWAS for extreme and early-onset obesity [7] , [12] , [54] , [55] , 11 showed directionally consistent association with BF% ( P binomal <0.006), of which five also reached nominal statistical significance ( Supplementary Table 25 ). Our meta-analysis of data from more than 100,000 individuals identified 12 loci significantly associated with BF%. While a recent GWAS including more than 340,000 individuals reported nearly 100 loci associated with BMI, a commonly used proxy measure for overall adiposity, four ( SPRY2 , IGF2BP1 , PLA2G6 and CRTC1 ) of the 12 BF% associated loci did not reach GWS for BMI, despite the enormous sample size [19] . This observation most likely reflects the heterogeneity of BMI as a marker of overall adiposity and emphasizes the increased statistical power of more precisely measured phenotypes. The 12 BF% associated loci divide into two distinct groups. The first group comprises the five loci ( FTO , MC4R , TMEM18 , SEC16B and SH2B1 ) of which the association is stronger with BMI than with BF%, suggesting that they affect both fat mass and lean mass. All five loci have been identified and described in detail before in relation with BMI [5] , [10] , [19] . Their associations with cardiometabolic outcomes are predictable, reflecting the phenotypic correlations with BF%; that is, their BF% increasing alleles are associated with an unfavourable glycemic and lipid profile and with an increased risk of T2D and CVD. The second group, comprising the remaining seven loci ( IRS1 , SPRY2 , TOMM40 / APOE , CRCT1 , PLA2G6 , IGB2BP1 and COBLL1 / GRB14 ), all show a more pronounced effect on BF% than on BMI, suggesting a specific effect on adiposity rather than on overall body mass. Most notably, the association patterns with cardiometabolic traits of this group of loci, as opposed to the first group, often do not reflect the phenotypic correlations. For example, as we have described before, the BF% increasing allele of the index SNP 500 kb upstream of IRS1 , which affects IRS1 expression, is associated with a favourable cardiometabolic risk profile, including a reduced risk of T2D and CVD [13] . We showed that this association signature, which goes against the phenotypic correlations, could be explained by an effect on fat distribution, as the BF% increasing allele was associated with increased subcutaneous, but not with the metabolically more harmful visceral fat [13] . The locus between GRB14 and COBLL1 shows a similar association signature. In fact, this locus was first described for its association with a lower WHR adjBMI [11] and reduced risk of T2D [30] . Here, we show that the same allele is associated with increased BF%, suggesting that the association with WHR adjBMI likely reflects a proportionally greater fat accumulation at hip and thighs rather than at the waist. Although this locus requires further experimental follow-up, current observations point towards GRB14 as the candidate gene in this locus. GRB14 encodes a protein that binds directly to the insulin receptor (IR), and the BF% increasing allele of the index SNP is associated with reduced GRB14 expression in adipose tissue. This is consistent with previous observations showing that Grb14/GRB14 expression is increased in adipose tissue of insulin-resistant rodents and in obese patients with T2D [56] . Furthermore, Grb14-deficient mice show improved glucose homeostasis and enhanced insulin action through increased IR-mediated IRS1 phosphorylation in the liver and skeletal muscle [57] . The similar cross-phenotype association signatures of the IRS1 and GRB14/COBLL1 loci might be a reflection of the close interaction between IRS1 and GRB14 in the IR-signalling pathway. The BF% increasing allele of the PLA2G6 locus is associated with lower insulin and TG levels and reduced T2D risk, particularly in men. PLA2G6 is the nearest gene and encodes a calcium-independent phospholipase A2 involved in the hydrolysis of phospholipids. However, this locus harbours a number of other genes that would make plausible candidates for driving the cross-phenotype associations, including PICK1 , which is membrane sculpting BAR domain protein. PICK1-deficient mice and flies display marked growth retardation, which at least in mice, might be due to impaired storage and secretion of growth hormone from the pituitary and possibly insulin from the pancreas [58] . PICK1-deficient mice, despite their smaller size, demonstrate increased body fat and reduced lean mass, reduced TG levels and impaired insulin secretion, which was compensated by increased insulin sensitivity [58] . Given the locus’ association with nevus count, SOX10, which encodes a member of the SOX (SRY-related HMG-box) family of transcription factors, is another candidate gene in this locus. SOX genes are involved in the regulation of embryonic development and SOX10 in particular is important for the development of neural crest and peripheral nervous system. Mutations in SOX10 have been implicated in uveal melanoma and Waardenburg syndrome, which presents with pigmentation abnormalities and hearing loss, and Kallmann syndrome, which presents with failure to start or complete puberty and hypogonadotropic hypogonadism (short stature, absence of puberty and sex hormones, among others) and absence of smell [59] , [60] . The phenotype similarity of these syndromes and the association signature may suggest that SOX10 could be driving the associations observed for the PLA2G6 locus. The TOMM40 / APOE locus is another locus with an intriguing association signature; while the BF% increasing allele has an unfavourable effect on glycemic traits and T2D risk, it is associated with a favourable lipid profile and reduced risk of CVD. The high LD in this region poses a major challenge to elucidate whether the association with lipid traits is due to a ‘spillover’ effect from nearby lipid-associated loci in APOE . Using conditional analyses, we provide evidence suggesting that at least the association with lower TG and high HDL-C levels might be distinct from previously reported loci. Of interest is that the BF% increasing allele seems to be associated with markers of increased longevity [41] . The CRTC1 locus is another gene-rich locus, but given the epigenetic marks in this gene and data from animal models, CRTC1 poses to be a good candidate gene. CRTC1 is primarily expressed in the brain, and it may affect leptin anorexic effect in the hypothalamus [61] . CRTC knockout mice demonstrated hyperphagia, increased white adipose tissue and infertility [61] . Our meta-analysis was limited by the fact that participating studies all had imputed HapMap reference panels for autosomal chromosomes and that the analysis model assumed additive effects. Future discovery efforts based on genome-wide imputation of 1000 Genomes reference panels, that include X- and Y-chromosomes and that also test recessive and dominant inheritance, will allow for the discovery of more and lower-frequency variants and for refining association signatures of already established BF%-associated loci. Taken together, our expanded genome-wide meta-analyses of BF% has identified a number of loci with distinct cross-phenotype association signature that, together with our functional follow-up analyses, facilitated the identification of strong positional candidates. Particularly striking is that two of the 12 loci harbour genes ( IRS1 , GRB14 ) that influence insulin receptor signalling, and two other loci contain genes ( IGF2BP1 , PICK1) that are involved in the GH/IGF1 pathway, that in turn also relates to insulin receptor signalling. Discovery of new loci Study design . A two-stage meta-analysis was performed to identify loci associated with BF%. In Stage 1, we conducted two parallel meta-analyses; one meta-analysis combined summary statistics from 43 GWAS, totalling up to 76,137 adult individuals (65,831 European ancestry, 7,557 South Asian ancestry, 2,333 East Asian ancestry and 416 African Americans), and the other meta-analysis combined summary statistics from 13 additional studies genotyped using the Metabochip, totalling up to 24,582 individuals (23,469 Europeans and 1,113 African Americans). In Stage 2, we combined the GWAS meta-analysis results and Metabochip meta-analysis results from Stage 1 ( Supplementary Table 1 and Supplementary Figs 1 and 2 ) in one final meta-analysis, including 100,716 individuals from 56 studies. All the studies were approved by their local institutional review boards and written consent was obtained from all the study participants. Although our primary analysis, described above, combined all the data available to us, in the secondary analyses, we conducted stratified analyses for (1) all-ancestry men-only, (2) all-ancestry women-only, (3) European ancestry, (4) European ancestry men-only and (5) European ancestry women-only ( Supplementary Tables 4–6 and Supplementary Figs 2–5 ). Phenotype . BF% in each cohort was measured either with bioimpedance analysis (BIA) or dual energy X-ray absorptiometry (DEXA) as described in detail before [13] . For each study, BF% was adjusted for age, age 2 and study-specific covariates (for example, genotype-based principle components, study centre and others), if necessary. For studies of unrelated individuals, the residuals were calculated separately in men and women, and in cases and controls. For studies of family-based design, the residuals were calculated in men and women together, and sex was additionally adjusted in the model. The residuals were then inverse normally transformed for association testing. For studies of family-based design, the family relatedness was additionally adjusted in the association testing. Sample quality control, imputation and association . Each study did the study-specific quality control (QC) ( Supplementary Table 2 ). The GWAS common SNPs were imputed in each study using the respective HapMap Phase II (Release 22) reference panels (EUR for studies of European-ancestry populations, CHB+JPT for studies of Eastern Asian ancestry populations, and CEU+YRI+CHB+JPT for studies of Indian Asian ancestry populations and African American populations). Individual SNPs were associated with inverse normally transformed BF% residuals using linear regression with an additive model. All the SNPs with low imputation scores (MACH r 2 -hat <0.3, IMPUTE proper_info <0.4 or PLINK info <0.8) and a MAC ≤3 were removed. The EasyQC software was used for detailed QC of study level analyses and meta-level analysis, as described elsewhere [62] . Meta-analysis . Meta-analyses were performed using inverse variance-weighted fixed-effect method in METAL. Inflation before genomic control (GC)-correction was generally low in all-ancestry ( λ men+women =1.13; λ men =1.07; λ women =1.09) and European-only ( λ men+women =1.13; λ men =1.07; λ women =1.10) analyses. To reduce the inflation of the test statistics from potential population structure, individual GWAS results and GWAS meta-analysis results were corrected for GC using all SNPs. Individual Metabochip results and Metabochip meta-analysis results were GC-corrected using 4,425 SNPs, which are derived from pruning of QT-interval replication SNPs within 500 kb of an anthropometry replication SNP on the Metabochip. The GC-corrected GWAS and Metabochip meta-analysis results were finally meta-analysed ( Supplementary Fig. 1 ). Using the LD score regression method in the European-only meta-analyses suggests that the observed inflation is not due to population substructure [63] . The regression intercept, which estimates inflation after removing polygenic signals, was 1.0045 (with λ GC =1.136 and mean χ 2 =1.16) for sex-combined, 0.999 ( λ GC =1.062 and mean χ 2 =1.079) for men-only and 1.014 ( λ GC =1.105 and mean χ 2 =1.112) for women-only analyses. Using these regression intercepts, rather than the λ GC , to correct our meta-analyses, results in more significant associations (for example, for the rs1558902- FTO SNP, P =3.24 × 10 −27 in the modified European sex-combined meta-analysis compared with P =1.1 × 10 −25 ( Supplementary Table 6 )). Overall, however, the less stringent correction did not result in the identification of novel loci. Identification of novel loci . Each unique locus was defined as ±500 kb on either side of the most significant SNP that reached a GWS threshold ( P <5 × 10 −8 ) in the meta-analysis. These GWS-index SNP loci from the primary analysis as well as from secondary analyses were highlighted for further analyses ( Table 1 and Supplementary Tables 4–6 ). The genotype data for the genome-wide significant SNPs was of high quality with a median imputation score of ≥0.95 ( Supplementary Table 26 ). The fifth percentile for all SNPs was ≥0.80, except for the previously established TOMM40 SNP (P5=0.52). Joint and conditional multiple SNP association analysis . We used the GCTA approach to identify potential additional signals in regions of GWS-index SNP. This approach uses summary meta-analysis statistics and a LD matrix from an ancestry-matched sample to perform approximate joint and conditional SNP association analysis. Although our primary analyses were based on all ancestry populations, the 12 GWS-index SNPs were strongly associated with BF% in European populations, 6 of them reaching the GWS ( Supplementary Table 5 ). The estimated LD matrix based on 6,654 unrelated individuals of European ancestry in ARIC cohort was used in the analysis. Heterogeneity among studies . The potential heterogeneity in the effect estimates for our GWS-index SNPs were investigated between men and women in all-ancestry populations and in European populations, and between individuals of European ancestry and individuals of all ancestry. We also tested for heterogeneity between results from studies that used BIA for BF% assessment and that used DEXA. Heterogeneity was assessed using a t -statistic, t =( β 1 − β 2 )/(se 1 2 +se 2 2 −2* r * se 1 *se 2 ) ½ to account for relatedness, where β 1 and β 2 are the effect size estimates, se 1 and se 2 are the corresponding standard errors and r is Spearman’s correlation coefficient of beta values between men and women or between European ancestry and all ancestry. Variance explained . The variance explained by each GWS-index SNP was calculated using the effect allele frequency ( f ) and beta ( β ) from the respective meta analyses using the formula [6] of Explained variance =2 f (1− f ) β 2 . Cross-trait association lookups Cardiometabolic consortia . To explore the relationship between BF% and an array of cardiometabolic traits and diseases, the association results for the 12 GWS-index SNPs were requested from seven primary cardiometabolic genetic consortia: the LEPgen consortium (circulating leptin, Kilpeläinen et al. , in preparation), VATGen consortium [27] , GIANT (BMI, height and WHR adjBMI ) [19] , [20] , [26] , GLGC (HDL-C, LDL-C, TG, TC) [28] , MAGIC [29] , DIAGRAM (T2D) [30] and CARDIoGRAMplusC4D (CAD) [31] . On the basis of known correlations among these cardiometabolic traits, we considered circulating leptin levels, abdominal adipose tissue storage, height, WHR adjBMI , plasma lipid levels, plasma glycemic traits, T2D and CAD as eight independent trait groups. In addition, the associations for these 12 SNPs were also looked up in four consortia that examined phenotypes more distantly related to BF%: ADIPOGen (BMI-adjusted adiponectin) [64] , ReproGen (age at menarche) [24] , liver enzyme meta-analysis [65] and CRP meta-analysis [38] . For certain GWAS-index SNPs, we also did specific lookups: rs6857 association in liver fat storage, rs3761445 associations in cutaneous nevi and melanoma risk meta-analysis [42] , [43] , [44] , early growth genetics (birth weight [32] and pubertal height [33] ), insulin-like growth factor 1 meta-analysis (Teumer et al. under review) and CHARGE testosterone meta-analysis [66] , and rs9906944 associations in tooth development meta-analysis [35] and Early Growth Genetics Consortium (birth weight [32] and pubertal height [33] ). NHGRI GWAS catalogue lookups . We manually curated and searched the National Human Genome Research Institute (NHGRI) GWAS Catalogue ( www.genome.gov/gwastudies ) for previously reported associations for SNPs within 500 kb and r 2 >0.7 (1000 Genomes Pilot1 EUR population based on SNAP: http://www.broadinstitute.org/mpg/snap/ldsearch.php ) with each of the 12 GWS-index SNPs. All previously reported associations that reached P <5 × 10 −8 were retained ( Supplementary Table 11 ). Coding variants and CNVs To determine whether any of our 12 GWS-index SNPs might be tagging potentially functional variants, we identified all variants within 500 kb and in LD ( r 2 >0.7, HapMap release 22/1000 Genomes Pilot1 EUR) with our GWS-index SNPs. As such, we identified 776 variants and annotated each of them using Annovar ( http://www.openbioinformatics.org/annovar/ ). The predicted functional impacts for coding variants were accessed via the Exome Variant Server ( http://evs.gs.washington.edu/EVS/ ) for PhastCon, Grantham, GERP and PolyPhen, and were also from SIFT ( http://sift.jcvi.org/ ). To determine whether any of the 12 GWS-index SNPs tagged ( r 2 >0.7) CNVs, all genetic variants (SNV, Indel and SVS) within a 1 Mb window of the index SNPs from the 1000 Genomes Project EUR population (Phase 1) were downloaded. The LD indexes were calculated between each of the 12 GWS-index SNPs and any nearby CNV variants. Analyses of eQTLs The cis -associations between 12 GWS-index SNPs and expression of nearby genes (±500 kb of the index-SNP) were examined in the whole blood ( n =2,360) from the eQTL meta-analysis study [67] , the abdominal fat tissue ( n =742 for omental fat and n =610 for subcutaneous fat) from the bariatric surgery study [68] , the abdominal subcutaneous fat tissue ( n =54) and gluteal subcutaneous fat tissue ( n =65) from the MolOBB study [69] , and the brain tissue from the cortical brain study ( n =193; ref. 70 ). Conditional analyses were conducted by including both GWS-index SNP and the most significant cis -associated SNP for the given transcript in the model to examine whether observed associations were driven by our GWS-index SNP or by other nearby variants. Conditional analyses were conducted for all tissues except the brain tissue. Regulatory annotation using ENCODE and Roadmap Regulatory element overlap . We identified variants in LD ( r 2 >0.7, 1000 Genomes Project Pilot, EUR) with each of the 12 GWS-index SNPs and tested for overlap between these variants and elements from regulatory datasets. In total, 746 variants at the 12 GWS-index loci were examined for overlap with regulatory elements in 181 data sets ( Supplementary Tables 18 and 19 ) from five tissues (blood, brain, liver, adipose tissue and pancreatic islets). These data sets, downloaded from the ENCODE Consortium and Roadmap Epigenomics Projects, identify regions of open chromatin (DNase-seq, FAIRE-seq), histone modification signal enrichment (H3K4me1, H3K27ac, H3K4me3, H3K9ac and H3K4me2), and transcription factor binding in cell lines and tissues believed to influence BF%. When available, we downloaded data processed as a part of the ENCODE Integrative Analysis. Roadmap Epigenomics sequencing data were processed with MACS2 and the same irreproducible discovery rate pipeline used in the ENCODE Integrative analysis when multiple data sets were available, or MACS2 alone when only a single replicate was available. Pol2 binding . We tested for correlation between Pol2 binding strength and genotype in lymphoblastoid cell lines at two SNPs, rs4808844 and rs4808845 that are in LD with GWS-index SNP of rs757318 in CRTC1 . Pol2 binding data uniformly processed as part of the ENCODE Integrative analysis were download for 10 lymphoblastoid cell lines (GM10847, GM12878, GM12891, GM12892, GM15510, GM18505, GM18526, GM18951, GM19099, GM19193). We examined the alleles present at these variants in Pol2 ChIP-seq alignment BAM files to determine sample genotypes and compared these with genotypes generated by the 1000 Genomes Project for the same samples. For the eight samples also genotyped by the 1000 Genomes Project, genotype calls were 100% concordant. Correlation between genotype and Pol2 binding signal at each SNP was calculated in R using a linear model (signal ∼ genotype). RegulomeDB annotation . We further characterized the variants at selected loci using the web-based tool RegulomeDB ( http://regulomedb.org/ ). The reference sequence identifiers of variants that overlap two or more regulatory elements in the same tissue were used to conduct the RegulomeDB search. Pathway, network and tissue-enrichment analysis To define pathways, networks and tissue enrichment, we extended the list of genome-wide significant loci to also include loci that showed putative ( P <1 × 10 −5 ) association with BF% (using the same criteria described above to define independent loci). As such loci, represented by 43 index SNPs, were considered for gene prioritization, pathway enrichment (DEPICT, Ingenuity Pathway Analyses), gene relationship analysis (GRAIL) and protein–protein interaction analyses (DAPPLE). Data-driven enrichment prioritized integration for complex traits . Details of this method are provided in Pers et al. [50] DEPICT is designed to systematically identify the most likely causal gene at a given locus, to test gene sets for enrichment for genetic associations, and to identify tissues and cell types in which genes from associated loci are highly expressed. DEPICT assigned genes to the 43 associated loci if the genes resided within the associated LD region ( r 2 >0.5) of a given associated SNP. After merging overlapping regions and discarding regions that mapped within the extended major histocompatibility complex locus, we were left with 42 non-overlapping regions that covered a total of 82 genes. We then used DEPICT to test enrichment at these loci for a total of 14,461 reconstituted gene sets, and for 209 tissue and cell type annotations. Ingenuity pathway analyses . We used HaploReg v2 ( http://www.broadinstitute.org/mammals/haploreg/haploreg.php ) and adopted a stringent LD ( r 2 >0.8 in 1000 Genome phase 1 EUR) to extract all the nearby genes (88 genes in total) of the index SNPs based on both GENCODE and RefSeq. For 65 out of them, they were successfully mapped to the Ingenuity Knowledge Base, and those unmapped genes are mainly lincRNA, miRNA, antisense or processed transcript genes derived from GENCODE. The 65 genes were incorporated into Ingenuity Canonical pathway enrichment analysis. The P values are calculated based on Fisher’s right-tailed exact test. The default settings were used for Ingenuity Interaction network analysis. Gene relationships among implicated loci . The GRAIL was used to examine relationships between genes. For each query and seed SNP, we adopted the default methods implemented in GRAIL to extract the genes around each index SNP: that is, (1) we first identified neighboring SNPs in the 3′ and 5′ direction in LD ( r 2 >0.5, CEU HapMap), proceeding outwards in each direction to the nearest recombination hotspots to define an interval region, and extracted all the genes in this interval; (2) if there are no genes in that interval region, the interval is extended an additional 250 kb in either direction. The 12 GWS-index SNP regions were input as seed regions, and the regions for the remaining 31 SNPs were input as query regions. Connections between genes were inferred from textual relationships based on published scientific text using PubMed abstracts as of December 2006. The significant gene similarity was declared based on P GRAIL <0.01. Disease association protein–protein link evaluator . The DAPPLE package was used to examine the potential encoded protein–protein interaction evidence for the genes located in the 43 associated loci. Genes from 32 of the 43 loci were annotated in the high-confidence pair-wise interaction InWeb database. Both the direct and indirect interactions were considered. The running settings were 1,000 permutation, common interactor binding degree =2, and 110 kb upstream and 40 kb downstream to define a gene’ residence. Drosophila knockdown experiments Genome-wide screen . We first identified all genes within ±500 kb of the 12 GWS-index SNPs, and subsequently identified the corresponding Drosophila orthologues available in the ensembl orthologue database ( www.ensembl.org , Supplementary Table 23 ). Drosophila triglyceride content values were mined from a publicly available genome-wide obesity screen data set [52] . Estimated values represent fractional changes in triglyceride content in adult male flies. Data are from male progeny resulting from crosses of male UAS-RNAi flies from the VDRC and Hsp70-GAL4; Tub-GAL8ts virgins females. Two-to-five-day-old males were sorted into groups of 20 and subjected to two 1-h wet heatshocks 4 days apart. On the seventh day, flies were picked in groups of eight, manually crushed and sonicated, and the lysates heat-inactivated for 10 min in a thermocycler at 95 °C. Centrifuge-cleared supernatants were then used for triglyceride (GPO Trinder, Sigma) and protein (Pierce) determination. Triglyceride values from these adult-induced ubiquitous RNAi knockdown individuals were normalized to those obtained in parallel from non-heatshocked progeny from the very same crosses. Targeted follow-up . Based on known biology, one to three potential candidate genes within ±500 kb of the 12 GWS-index SNPs were selected. Corresponding Drosophila orthologues were available for 11 loci, but no orthologue exists for FTO ( Supplementary Table 24 , http://www.flyrnai.org/cgi-bin/DRSC_orthologs.pl ). The respective fly RNAi stocks for each Drosophila orthologue were acquired from the Vienna Drosophila Resource Center, as well as genetic background controls w1118 (for GD lines, VDRC #60000); tub-gal4/TM6 and w; tub-gal80ts/TM6 is available from the Bloomington Drosophila Stock Center. For fly triglyceride assay in the adult, male RNAi flies were crossed with w; tub-gal4 tub-gal80ts/TM6 virgins. Progenies were kept in 16 °C until enclosure. Adults were transferred to 25 °C for 2 weeks. Whole-animal triglycerides were measured as previously described [53] . Briefly, triglycerides were measured using the Infinity Triglycerides Reagent kit (Thermo Fisher #TR22321) on whole-animal homogenates of groups of three animals. Proteins from the same homogenates were measured using the Pierce BCA protein Assay kit (Thermo Scientific #23227). Triglycerides were normalized by proteins. Data were average of three experiments. The fractional changes in triglyceride content in adult male flies between knockdown group and the control groups were compared using the two-tailed t -tests in SAS version 9.2 software (SAS Institute, Cary, NC). How to cite this article: Lu, Y. et al. New loci for body fat percentage reveal link between adiposity and cardiometabolic disease risk. Nat. Commun. 7:10495 doi: 10.1038/ncomms10495 (2016).